Folding of Toll-like receptors by the HSP90 paralogue gp96 requires a substrate-specific cochaperone Cytosolic HSP90 requires multiple cochaperones in folding client proteins. However, the function of gp96 (HSP90b1, grp94), an HSP90 paralogue in the endoplasmic reticulum (ER), is believed to be independent of cochaperones. Here, we demonstrate that gp96 chaperones multiple Toll-like receptors (TLRs), but not TLR3, in a manner that is dependent on another ER luminal protein, CNPY3. gp96 directly interacts with CNPY3, and the complex dissociates in the presence of adenosine triphosphate (ATP). Genetic disruption of gp96–CNPY3 interaction completely abolishes their TLR chaperone function. Moreover, we demonstrate that TLR9 forms a multimolecular complex with gp96 and CNPY3, and the binding of TLR9 to either molecule requires the presence of the other. We suggest that CNPY3 interacts with the ATP-sensitive conformation of gp96 to promote substrate loading. Our study has thus established CNPY3 as a TLR-specific cochaperone for gp96. Gp96 is the endoplasmic reticulum (ER) resident member of the HSP90 family. Known also as grp94, HSPC4 (ref. 1 ) or HSP90b1 (ref. 2 ), gp96 has an intrinsic ATPase activity [3] , [4] , [5] and it shares ∼ 50% homology with the cytosolic HSP90 at the amino-acid level, consisting of the N-terminal adenosine triphosphate (ATP)-binding domain (N), followed by the charged middle domain (M) and the C-terminal homodimerization domain (C). It is constitutively expressed in virtually all cell types and its expression is upregulated by stress conditions that perturb ER functions [6] . HSP90 can chaperone up to 10% of the proteome [7] , [8] , and its function is assisted by a number of well-characterized cochaperones such as Hop, p23, Aha1 and CDC37 (ref. 9 ). These cochaperones modulate the ability of HSP90 to interact with its substrates and ATP, which are critical for the proper and necessary conformational changes of HSP90, including N-domain dimerization, in order to complete the cycle of substrate binding and release. Recently, gp96 has been found to be a master chaperone for multiple Toll-like receptors (TLRs) and integrins [10] , [11] , [12] , [13] . Deletion of gp96 in either macrophages or B cells resulted in inactivation of multiple TLRs at the post-translational level. However, it remains unclear whether gp96 chaperones its client proteins alone or does so in concert with unidentified cochaperones. The prevailing idea has been that gp96 is a unique member of the HSP90 family in that it does not require a cochaperone for function [14] . Consistent with this notion is that gp96 does not share the common structural features with HSP90, such as the C-terminal methionine-glutamic acid-glutamic acid-valine-aspartic acid motif for binding to cochaperones. Yet, the structural study of the near full-length gp96 (NMC) clearly suggests that additional factors are necessary for N-domain dimerization of gp96, leading to optimal function [5] . The 'extended-open' form of the N and M domains of the gp96 dimer in the presence of ADP and adenylyl-imidodiphosphate (AMP-PNP) is incompatible with its chaperone function [5] . TLRs are a family of pattern recognition receptors for pathogens that have critical roles in innate immunity against infection [15] . Thirteen TLRs exist in mammals and they localize either on the cell surface or in the endolysosome compartment. Surface TLRs, including TLR1, TLR2, TLR4, TLR5, TLR6 and TLR11, primarily recognize microbial non-nucleic acid structures. In contrast, intracellular TLRs recognize nucleic acid-based molecules: TLR3 for double-stranded RNA (dsRNA), TLR7/8 for single-stranded RNA and TLR9 for DNA. All TLRs are type I transmembrane (tm) receptors sharing characteristic structural features: an N-terminal ectodomain containing multiple leucine-rich repeats (LRRs) for ligand binding, a short helix embedded in the membrane and a C-terminal cytosolic tail containing the Toll-interleukin (IL)-1 receptor domain for recruiting signalling adaptors. TLR9 resides in the ER in the steady state. It has to exit from the ER by binding to the membrane protein Unc93b (ref. 16 ), and is further matured by a proteolytic cleavage of the first 14 N-terminal LRRs [17] , [18] in the endolysosomal compartment where signals originate [19] . TLR9 binds to a diverse range of DNA sequences [20] , which induces a conformational change of the ectodomain and the close apposition of the dimeric cytoplasmic signalling tails [21] . TLR3 is a pattern recognition receptor for dsRNA produced commonly as the viral replication intermediate [22] . Activation of TLR3 also occurs in the acidic endosomal location [23] . Unlike all other TLRs that can signal through MyD88, the signalling of TLR3 depends exclusively on the cytosolic adaptor molecule TRIF [24] . Murine canopy3 (CNPY3) (UniProt accession: Q9DAU1 ) is a ubiquitous ER luminal protein of ∼ 35 kDa [25] . CNPY3 has a unique pattern of six cysteine residues [26] , which is characteristic of the saposin-like proteins that form a shell-like dimer [27] . It also has a C-terminal basic region formed by a stretch of lysine-rich repeat. Although CNPY3 was initially thought to be important for TLR4 expression and was also named PRAT4A (a protein interacting with TLR4) [28] , cnpy3 knockout (KO) mice lost the function of multiple TLRs post-translationally, except TLR3 (ref. 25 ). In this study, we demonstrate that CNPY3 and gp96 depend on each other for post-translational maturation of multiple TLRs, except TLR3. CNPY3 and gp96 form a complex both in vitro and in vivo . The interaction between these two molecules is critical for TLR9 folding and transport to the endolysosomes. We conclude that CNPY3 is the elusive TLR-specific cochaperone of gp96. Furthermore, we propose a model in which CNPY3 interacts with the ATP-sensitive conformation of the gp96 N domain to keep the overall structure of gp96 in the relaxed state in order to facilitate the 'loading' of TLRs onto gp96 for completion of the folding cycle. gp96 and CNPY3 are dispensable for TLR3 function There are multiple dsRNA sensors in the cell, including the endosomal TLR3 and the cytosolic retinoic acid-inducible gene I, melanoma differentiation-associated gene 5 and protein kinase R [29] . We first performed a series of studies to resolve the role of gp96 in TLR3 function. We found that gp96 KO peritoneal macrophages (pMφ) produced high levels of IL-6 and tumour-necrosis factor-α ( Fig. 1a ) after stimulation with a synthetic dsRNA analogue polyI:C [30] . The responsiveness of pMφ to polyI:C was mediated by TLR3 but not by TLR2 or TLR4, as it was abrogated in tlr3 −/− pMφ, but preserved in tlr2 −/− tlr4 −/− double KO cells. In addition, we found that gp96 KO B cells [12] upregulated surface CD69 shortly after polyI:C stimulation, which was strictly dependent on TLR3 (ref. 22 ) ( Fig. 1b ). We also examined whether the function of enforced expression of TLR3 required gp96, using a gp96 mutant pre-B-cell line that stably expresses a nuclear factor-κB-green fluorescent protein reporter [11] . Neither wild-type (WT) nor mutant (Mut) pre-B cells responded to polyI:C without enforced TLR3 expression ( Fig. 1c ). However, transfection with TLR3, but not with TLR9 expression vector, rendered both WT and Mut cells responsive. These cells express endogenous TLR9; overexpression of TLR9HA does not rescue CpG responsiveness of Mut cells ( Supplementary Fig. S1 ). Taken together, we conclude that TLR3 folding is independent of gp96. Thus, gp96 KO cells phenocopy the TLR defects of CNPY3 KO cells [25] . 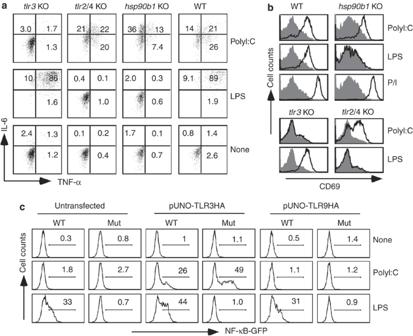Figure 1: gp96 is dispensable for TLR3 function. (a) Peritoneal Mφ fromtlr3−/−,tlr2−/−tlr4−/−,hsp90b1knockout (KO) and control mice were stimulated with polyI:C (100 μg ml−1), lipopolysaccharide (LPS) (1 μg ml−1) or medium (none) in the presence of brefeldin A (BFA) for 6 h. Cells were then stained and analysed for intracellular cytokine by flow cytometry. Numbers represent the percentage of cells in each quadrant over the total number of cells analysed. (b) Purified CD19+splenic-B cells from various mice were stimulated with polyI:C (100 μg ml−1), LPS (1 μg ml−1) or phorbol 12-myristate-13-acetate and ionomycin (P/I) for 6 h. Cells were then analysed for surface CD69 by flow cytometry. Open histograms represent CD69 stain and shaded histograms are isotype controls. (c) pUNO-TLR3HA or pUNO-TLR9HA expression vectors were introduced into WT and gp96 mutant pre-B cells. Cells were stimulated with polyI:C (100 μg ml−1) or LPS (1 μg ml−1) for 12 h, before flow cytometric analysis for nuclear factor-κB-driven green fluorescent protein (GFP). Numbers represent % of GFP+cells. Three experiments were conducted with similar results. Figure 1: gp96 is dispensable for TLR3 function. ( a ) Peritoneal Mφ from tlr3 −/− , tlr 2 −/− tlr4 −/− , hsp90b1 knockout (KO) and control mice were stimulated with polyI:C (100 μg ml −1 ), lipopolysaccharide (LPS) (1 μg ml −1 ) or medium (none) in the presence of brefeldin A (BFA) for 6 h. Cells were then stained and analysed for intracellular cytokine by flow cytometry. Numbers represent the percentage of cells in each quadrant over the total number of cells analysed. ( b ) Purified CD19 + splenic-B cells from various mice were stimulated with polyI:C (100 μg ml −1 ), LPS (1 μg ml −1 ) or phorbol 12-myristate-13-acetate and ionomycin (P/I) for 6 h. Cells were then analysed for surface CD69 by flow cytometry. Open histograms represent CD69 stain and shaded histograms are isotype controls. ( c ) pUNO-TLR3HA or pUNO-TLR9HA expression vectors were introduced into WT and gp96 mutant pre-B cells. Cells were stimulated with polyI:C (100 μg ml −1 ) or LPS (1 μg ml −1 ) for 12 h, before flow cytometric analysis for nuclear factor-κB-driven green fluorescent protein (GFP). Numbers represent % of GFP + cells. Three experiments were conducted with similar results. Full size image gp96 forms a complex with CNPY3 in multiple cell types Given the remarkable similarities of TLR phenotypes between gp96 and CNPY3 KO mice [10] , [25] , we suspected that CNPY3 might be a cochaperone of gp96 for TLR folding. If so, gp96 should bind to CNPY3. We addressed this prediction in multiple cell types. We found that gp96 and CNPY3 colocalize with each other intracellularly ( Fig. 2a ). Both proteins are localized in the ER as identified by an ER marker calnexin (CNX) but not with a lysosomal marker lysosomal-associated membrane protein-2 ( Supplementary Fig. S2 ). More important, gp96 coimmunoprecipitates with the endogenous CNPY3 in Raw264.7 macrophages and primary bone marrow-derived macrophages ( Fig. 2b ). We also observed that gp96 forms a complex with the C-terminal FLAG-tagged CNPY3 (CNPY3-FLAG) in HEK293 cells ( Fig. 2c ) and pre-B cells ( Fig. 2d ). By generating deletion mutants of gp96, we further showed that the first 355 amino acids of the N domain and part of the M domain of gp96 (N355) were sufficient to interact with CNPY3 ( Fig. 2e ). The C-terminal domain of gp96 (C150) does not interact with CNPY3 ( Fig. 2e ). 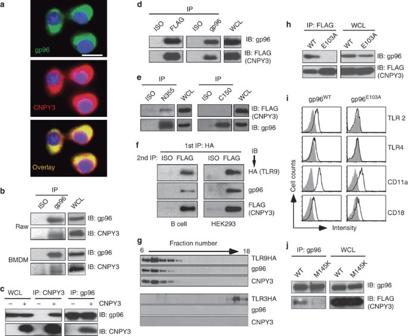Figure 2: gp96 forms a functionally significant complex with CNPY3 in multiple cell types. (a) Colocalization of gp96 with CNPY3-FLAG in Raw 264.7 macrophages by immunofluorescence microscopy after costaining with antibody against gp96 and FLAG. Scale bar, 20 μm. (b) gp96 was immunoprecipitated (IP) from Raw 264.7 macrophages or bone marrow-derived macrophages (BMDMs), followed by immunoblot (IB) for gp96 and endogenous CNPY3. (c) HEK293 cells were mock transfected or transfected with CNPY3-FLAG. After 48 h, cells were immunoprecipitated with FLAG or gp96 antibody, resolved on SDS–PAGE and immunoblotted for gp96 and FLAG. As a control, whole-cell lysates (WCLs) were also blotted for CNPY3 and gp96. (d) WT pre-B cells were immunoprecipitated for CNPY3-FLAG or gp96, or with isotype (ISO) control antibody, followed by IB for CNPY3 and gp96. (e) IP of N-fragment of gp96 (N355) or C-fragment of gp96 (C150) from mutant pre-B cells, followed by IB for CNPY3-FLAG and gp96. (f) Sequential IP analysis for TLR9–gp96–CNPY3 interaction in pre-B and HEK293 cells. IP of TLR9-HA, followed by elution with HA peptide, re-IP with FLAG antibody for CNPY3-FLAG and IB for indicated molecules. (g) IP of TLR9HA or TLR3HA from pre-B cells, followed by elution with HA peptide, gel filtration on Superdex 200 column and IB identification of proteins in indicated fractions. (h) IP of gp96 or gp96E103Amutant from pre-B cells expressing the respective proteins, followed by IB for CNPY3-FLAG and gp96. (i) gp96-null pre-B cell lines were spin-infected with MigR1-gp96E103Aor MigR1-gp96WTretroviral vectors, followed by staining of various gp96 client proteins on cell surface and flow cytometric analysis. (j) Raw 264.7 cells were transfected with WT CNPY3 or mutant CNPY3 (M145K). IP of gp96 was performed, followed by IB for CNPY3-FLAG or gp96. Results were confirmed by multiple experiments. Figure 2: gp96 forms a functionally significant complex with CNPY3 in multiple cell types. ( a ) Colocalization of gp96 with CNPY3-FLAG in Raw 264.7 macrophages by immunofluorescence microscopy after costaining with antibody against gp96 and FLAG. Scale bar, 20 μm. ( b ) gp96 was immunoprecipitated (IP) from Raw 264.7 macrophages or bone marrow-derived macrophages (BMDMs), followed by immunoblot (IB) for gp96 and endogenous CNPY3. ( c ) HEK293 cells were mock transfected or transfected with CNPY3-FLAG. After 48 h, cells were immunoprecipitated with FLAG or gp96 antibody, resolved on SDS–PAGE and immunoblotted for gp96 and FLAG. As a control, whole-cell lysates (WCLs) were also blotted for CNPY3 and gp96. ( d ) WT pre-B cells were immunoprecipitated for CNPY3-FLAG or gp96, or with isotype (ISO) control antibody, followed by IB for CNPY3 and gp96. ( e ) IP of N-fragment of gp96 (N355) or C-fragment of gp96 (C150) from mutant pre-B cells, followed by IB for CNPY3-FLAG and gp96. ( f ) Sequential IP analysis for TLR9–gp96–CNPY3 interaction in pre-B and HEK293 cells. IP of TLR9-HA, followed by elution with HA peptide, re-IP with FLAG antibody for CNPY3-FLAG and IB for indicated molecules. ( g ) IP of TLR9HA or TLR3HA from pre-B cells, followed by elution with HA peptide, gel filtration on Superdex 200 column and IB identification of proteins in indicated fractions. ( h ) IP of gp96 or gp96 E103A mutant from pre-B cells expressing the respective proteins, followed by IB for CNPY3-FLAG and gp96. ( i ) gp96-null pre-B cell lines were spin-infected with MigR1-gp96 E103A or MigR1-gp96 WT retroviral vectors, followed by staining of various gp96 client proteins on cell surface and flow cytometric analysis. ( j ) Raw 264.7 cells were transfected with WT CNPY3 or mutant CNPY3 (M145K). IP of gp96 was performed, followed by IB for CNPY3-FLAG or gp96. Results were confirmed by multiple experiments. Full size image If gp96–CNPY3 interaction is functionally required for TLR folding, two predictions can be made. First, TLR must interact with gp96–CNPY3 to form a trimolecular complex during the folding process. Second, abrogation of gp96–CNPY3 interaction should lead to defective TLR folding. Using TLR9 as a substrate, we found that both of these two predictions were correct. We expressed a C-terminal haemagglutinin (HA) epitope-tagged TLR9 in pre-B cells that coexpress gp96 and CNPY3-FLAG. We subjected the cells to treatment with a thiocleavable crosslinker, dithiobis succinimidyl propionate, to maintain tertiary stable complexes before immunoprecipitation for TLR9HA. The immunoprecipitates were then eluted with HA peptide, followed by either reimmunoprecipitation for CNPY3 or gel filtration analysis. The final product was identified by immunoblot for TLR9, CNPY3 and gp96. The sequential immunoprecipitation analysis indeed demonstrated that TLR9 forms a molecular complex with both CNPY3 and gp96 ( Fig. 2f ), which was confirmed by coelution of all three proteins from the gel filtration column ( Fig. 2g ). Consistent with no roles of gp96 or CNPY3 in TLR3 folding, similar analysis failed to demonstrate any interaction between TLR3 and gp96/CNPY3 ( Fig. 2g ). We next performed mutagenesis to determine the influence of loss of gp96–CNPY3 interaction on their ability to fold TLR9. We found that a single point mutation of gp96 at amino acid 103 (Glu) (gp96 E103A ) knocked down its ability to interact with CNPY3 ( Fig. 2h ), which correlated with the loss of chaperone function for TLRs but not for integrins ( Fig. 2i ). Similarly, we found that the loss-of-function variant CNPY3 M145K (ref. 31 ) was unable to interact with gp96 ( Fig. 2j ). Taken together, we concluded that gp96–CNPY3 interaction is critical for folding TLR9. CNPY3 binds to gp96 directly To determine whether gp96 directly interacts with CNPY3, we performed an in vitro binding assay between purified mouse gp96 and recombinant C-terminal GST (glutathione- S -transferase)-tagged CNPY3 (CNPY3-GST) ( Fig. 3a ). We found that gp96 was able to directly interact with both soluble ( Fig. 3b ) and immobilized CNPY3-GST but not with control protein GST ( Fig. 3c ). As HSP90 cochaperones are known to modulate the ATP-binding properties of HSP90, we examined the effect of ATP on CNPY3–gp96 interaction. We found that ATP dose-dependently inhibited the binding of gp96 to CNPY3 ( Fig. 3d ). ATP hydrolysis was not critical for such an inhibition, as the association between gp96 and CNPY3 could be prevented by a non-hydrolysable ATP analogue AMP-PNP ( Fig. 3d ), as well as by ADP ( Fig. 3e ). CNPY3 has neither intrinsic ATPase activity nor the ability to significantly modulate the ATPase activity of gp96 ( Supplementary Fig. S3 ). These data, in conjunction with the fact that the ATP-binding mutant gp96 E103A was unable to interact with CNPY3, suggest that CNPY3 binds to the adenosine nucleotide-sensitive N domain of gp96. 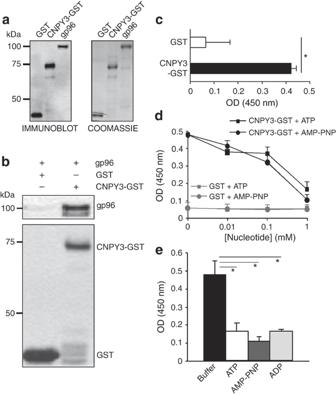Figure 3: gp96 directly interacts with CNPY3. (a) Characterization of gp96, recombinant GST and CNPY3-GST by immunoblot and coomassie blue staining after resolution on 10% sodium dodecyl sulphate–polyacrylamide gel electrophoresis (SDS–PAGE). (b) GST or CNPY3-GST was preincubated with glutathione beads, followed sequentially by blocking with bovine serum albumin (BSA) and incubation with gp96 for 2 h. The pulldown materials were immunoblotted for gp96 or GST as indicated. (c) Plate-bound GST or CNPT3-GST was incubated with gp96, followed by washing, blocking with BSA and detection of bound gp96 with ELISA in duplicates. Data are means of five independent experiments, error bars indicate standard error of mean. *P0.05. (d) and (e) Effect of adenosine nucleotide on gp96-CNPY3 interaction. Same as in (c), except that various inhibitors at the titrated dose (d) or 1 mM (e) were present during incubation with gp96 (10 μg ml−1). Data points are means of three individual experiments. Assays were performed in duplicates. Error bars indicate standard error of mean. *P<0.05. Figure 3: gp96 directly interacts with CNPY3. ( a ) Characterization of gp96, recombinant GST and CNPY3-GST by immunoblot and coomassie blue staining after resolution on 10% sodium dodecyl sulphate–polyacrylamide gel electrophoresis (SDS–PAGE). ( b ) GST or CNPY3-GST was preincubated with glutathione beads, followed sequentially by blocking with bovine serum albumin (BSA) and incubation with gp96 for 2 h. The pulldown materials were immunoblotted for gp96 or GST as indicated. ( c ) Plate-bound GST or CNPT3-GST was incubated with gp96, followed by washing, blocking with BSA and detection of bound gp96 with ELISA in duplicates. Data are means of five independent experiments, error bars indicate standard error of mean. * P 0.05. ( d ) and ( e ) Effect of adenosine nucleotide on gp96-CNPY3 interaction. Same as in ( c ), except that various inhibitors at the titrated dose ( d ) or 1 mM ( e ) were present during incubation with gp96 (10 μg ml −1 ). Data points are means of three individual experiments. Assays were performed in duplicates. Error bars indicate standard error of mean. * P <0.05. Full size image CNPY3 is required for gp96 to chaperone TLR9 We next addressed the roles of CNPY3 in the ability of gp96 to chaperone TLR9. We knocked down CNPY3 using a short hairpin RNA (shRNA) lentiviral vector. This strategy effectively silenced CNPY3, as evidenced by significant reduction of CNPY3 mRNA ( Fig. 4a ), cell surface TLR4 expression ( Fig. 4b ), as well as functional loss of multiple TLRs including TLR2, TLR4, TLR7 and TLR9 ( Fig. 4c,d ). Moreover, consistent with the idea that only fully folded TLR9 proceeds from the ER to the endolysosome for further proteolytic cleavage in this compartment [17] , [18] , CNPY3 silencing resulted in loss of the mature, cleaved form of TLR9 (TLR9 m, ∼ 80 kDa, Fig. 4e ). The expression level and stability of gp96 or full-length TLR9 were unaffected by CNPY3 interference ( Fig. 4e,f ), suggesting that CNPY3 is not the chaperone of gp96 per se . We next performed coimmunoprecipitation analysis to determine whether CNPY3 reduction affects the interaction between gp96 and TLR9. We were able to pull down similar levels of gp96 from control and CNPY3 shRNA-treated cells with gp96 antibody. However, gp96-associated TLR9 was significantly reduced in the absence of CNPY3 ( Fig. 4f ). Similar results were obtained using a small interfering RNA oligo (siRNA) that targets a different region of CNPY3 ( Fig. 4f ). We thus concluded that CNPY3 facilitates gp96 to chaperone TLR9, perhaps by locking ATP-free gp96 in a relaxed state for TLR9 loading. 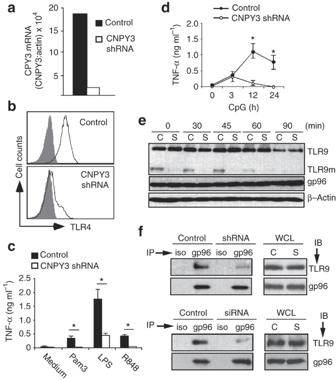Figure 4: CNPY3 promotes gp96–TLR9 interaction. (a) CNPY3 mRNA level (mean of duplicates) by a quantitative-PCR (Q-PCR) analysis after CNPY3 short-hairpin RNA (shRNA) interference. (b) Surface TLR4 expression (open histogram) on Raw264.7 cells after shRNA knockdown of CNPY3. Shaded histograms represent staining with isotype control antibody. (c) CNPY3 or control shRNA lentivirus-transduced Raw264.7 cells were stimulated with various TLR ligands for 3 h (Pam3 100 ng ml−1; lipopolysaccharide 200 ng ml−1, R848 50 ng ml−1), followed by measurement of tumour-necrosis factor-α in the supernatant by ELISA. All assays were performed in duplicates. Data are means of three independent experiments, error bar indicates standard error of mean. *P<0.05. (d) Same as (c), except that cells were stimulated with CpG (1 μM) for indicated times. Data points are means of three independent experiments. (e) Total cell lysates were incubated at 37°C for indicated time and blotted for TLR9HA and gp96 in cells transduced with CNPY3 (S) or control (C) shRNA lentiviral vector. (f) gp96 IP was performed using cells in (e) (top panel), or cells pretreated with CNPY3 siRNA (bottom panel), followed by IB for TLR9HA and gp96. Protein expression in whole-cell lysate is also shown. Figure 4: CNPY3 promotes gp96–TLR9 interaction. ( a ) CNPY3 mRNA level (mean of duplicates) by a quantitative-PCR (Q-PCR) analysis after CNPY3 short-hairpin RNA (shRNA) interference. ( b ) Surface TLR4 expression (open histogram) on Raw264.7 cells after shRNA knockdown of CNPY3. Shaded histograms represent staining with isotype control antibody. ( c ) CNPY3 or control shRNA lentivirus-transduced Raw264.7 cells were stimulated with various TLR ligands for 3 h (Pam3 100 ng ml −1 ; lipopolysaccharide 200 ng ml −1 , R848 50 ng ml −1 ), followed by measurement of tumour-necrosis factor-α in the supernatant by ELISA. All assays were performed in duplicates. Data are means of three independent experiments, error bar indicates standard error of mean. * P <0.05. ( d ) Same as ( c ), except that cells were stimulated with CpG (1 μM) for indicated times. Data points are means of three independent experiments. ( e ) Total cell lysates were incubated at 37°C for indicated time and blotted for TLR9HA and gp96 in cells transduced with CNPY3 (S) or control (C) shRNA lentiviral vector. ( f ) gp96 IP was performed using cells in ( e ) (top panel), or cells pretreated with CNPY3 siRNA (bottom panel), followed by IB for TLR9HA and gp96. Protein expression in whole-cell lysate is also shown. Full size image The chaperone function of CNPY3 is dependent on gp96 To gauge the roles of gp96 in CNPY3 function, we attenuated gp96 expression in macrophages by gp96 shRNA. We found that CNPY3 expression is not compromised by the reduction of gp96 ( Fig. 5a ). Similar to the defect of TLR9 cleavage in single CNPY3 knockdown cells, we found that TLR9 cleavage failed to occur in the absence of gp96 ( Fig. 5b ). Furthermore, on the basis of the differential sensitivity to endoglycosidase Endo H and PNGase F, and the fact that TLR9 cleavage occurs in the endolysosome, we found that TLR9 precursors were trapped in the ER of cells with silenced expression of either gp96 or CNPY3 ( Fig. 5b ). We next examined the roles of gp96 in CNPY3–TLR9 interaction in WT and gp96 KO pre-B cells. We found no difference in the expression of CNPY3 or TLR9 between these two cell types ( Fig. 5c ). However, the cooperative roles of gp96 and CNPY3 in TLR9 folding suggest that CNPY3 alone is unable to efficiently chaperone TLR9. To address this hypothesis, we compared the level of the CNPY3–TLR9 complex in gp96 WT and KO B cells. We found that both TLR9 and gp96 could be pulled down, along with CNPY3, in WT cells, but the amount of TLR9 that was coprecipitated with CNPY3 was significantly reduced in gp96 KO cells ( Fig. 5d ). Similarly, very little CNPY3 was coprecipitated with TLR9 in the absence of gp96 ( Fig. 5e ). Taken together, our data demonstrated that gp96 and CNPY3 are dependent on each other for TLR9 binding, which is consistent with a model that CNPY3 facilitates TLR9 loading to free gp96. 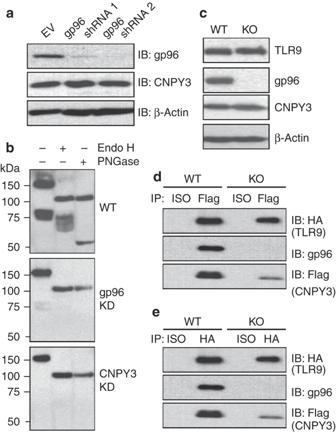Figure 5: CNPY3–TLR9 interaction is dependent on gp96. (a) Expression of endogenous CNPY3 and gp96 by Raw264.7 after transduction with empty vector (EV), and one or two rounds of gp96 shRNA lentivector. β-Actin is shown as a loading control. (b) Lack of cleaved form of TLR9 (TLR9 m) in the absence of gp96 or CNPY3. Total lysates of wild-type (WT) Raw264.7, cells that were knocked down (KD) for gp96 (gp96 KD) or CNPY3 (CNPY3 KD) were untreated, or treated with Endo H or PNGase F, followed by IB for TLR9HA. (c) WT or gp96 Mut pre-B cells were immunoblotted for TLR9-HA, gp96, CNPY3-FLAG and β-actin. (d) IP of CNPY3 from WT or gp96 KO cells, followed by IB for indicated proteins. (e) IP of TLR9-HA from WT or gp96 KO cells, followed by IB for indicated proteins. ISO indicated IP with isotype control antibody. Two experiments were conducted with similar results. Figure 5: CNPY3–TLR9 interaction is dependent on gp96. ( a ) Expression of endogenous CNPY3 and gp96 by Raw264.7 after transduction with empty vector (EV), and one or two rounds of gp96 shRNA lentivector. β-Actin is shown as a loading control. ( b ) Lack of cleaved form of TLR9 (TLR9 m) in the absence of gp96 or CNPY3. Total lysates of wild-type (WT) Raw264.7, cells that were knocked down (KD) for gp96 (gp96 KD) or CNPY3 (CNPY3 KD) were untreated, or treated with Endo H or PNGase F, followed by IB for TLR9HA. ( c ) WT or gp96 Mut pre-B cells were immunoblotted for TLR9-HA, gp96, CNPY3-FLAG and β-actin. ( d ) IP of CNPY3 from WT or gp96 KO cells, followed by IB for indicated proteins. ( e ) IP of TLR9-HA from WT or gp96 KO cells, followed by IB for indicated proteins. ISO indicated IP with isotype control antibody. Two experiments were conducted with similar results. Full size image gp96 and CNPY3 chaperone the ectodomain of multiple TLRs TLR molecules are sorted to different subcellular compartments through localization signals in the tm region and cytosolic tail of TLRs [32] , [33] , [34] . As both CNPY3 and gp96 reside in the ER lumen, we hypothesized that gp96 and CNPY3 assist the folding of ectodomains of TLRs, except that of TLR3. To directly address this hypothesis, we generated a TLR fusion protein that contains the ectodomain of TLRs and the tm domain of the platelet-derived growth factor receptor ( Fig. 6a ) [35] , [36] . The tm domain and the entire cytoplasmic tail of TLRs were deleted to avoid the potential impact of cytoplasmic signalling tails on cell surface expression of TLR fusion proteins. We reasoned that surface expression of these fusion TLRs is a good indication of their folding status, as misfolded proteins would not be allowed to exit ER because of the well-known ER protein quality control mechanism [37] . 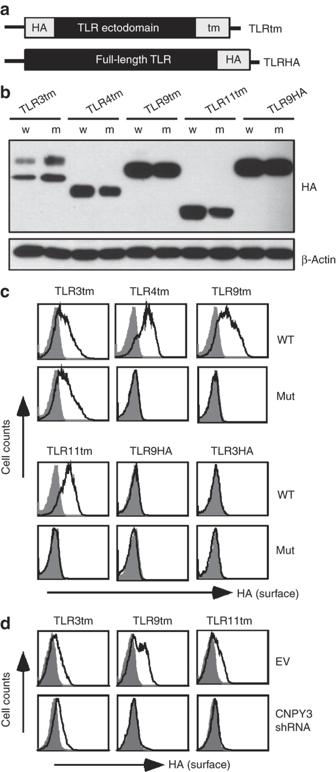Figure 6: gp96 and CNPY3 chaperone the ectodomains of multiple TLRs, but not that of TLR3. (a) Schematic diagram of TLR fusion proteins. HA represents haemagglutinin epitope from the influenza virus. The transmembrane domain of the platelet-derived growth factor (PDGF) receptor is indicated as tm. Signal peptide is not depicted. (b) TLR fusion proteins are detected by HA immunoblotting from retroviral transduced pre-B cells (w-WT, m-Mut cells). TLR3 doublets represent difference in N-linked glycosylation. β-actin is probed as a loading control. (c) WT and gp96 mutant (mut) pre-B cells were transduced with indicated retrovirus, followed by flow cytometric analysis of surface TLR with HA antibody (open histogram). Shaded histograms are staining controls with isotype-matched antibody. Multiple experiments were conducted with similar results. (d) Empty vector (EV) and CNPY3-silenced Raw264.7 cells were transduced with various TLRtm vectors, followed by cell surface staining of TLRtms (open histogram). Shaded histogram represents staining with untransduced cells. Figure 6: gp96 and CNPY3 chaperone the ectodomains of multiple TLRs, but not that of TLR3. ( a ) Schematic diagram of TLR fusion proteins. HA represents haemagglutinin epitope from the influenza virus. The transmembrane domain of the platelet-derived growth factor (PDGF) receptor is indicated as tm. Signal peptide is not depicted. ( b ) TLR fusion proteins are detected by HA immunoblotting from retroviral transduced pre-B cells (w-WT, m-Mut cells). TLR3 doublets represent difference in N-linked glycosylation. β-actin is probed as a loading control. ( c ) WT and gp96 mutant (mut) pre-B cells were transduced with indicated retrovirus, followed by flow cytometric analysis of surface TLR with HA antibody (open histogram). Shaded histograms are staining controls with isotype-matched antibody. Multiple experiments were conducted with similar results. ( d ) Empty vector (EV) and CNPY3-silenced Raw264.7 cells were transduced with various TLRtm vectors, followed by cell surface staining of TLRtms (open histogram). Shaded histogram represents staining with untransduced cells. Full size image As expected, there was no cell surface expression of either TLR9HA or TLR3HA in WT or Mut cells ( Fig. 6c ). Interestingly, TLRtms (TLR3tm, TLR4tm, TLR9tm and TLR11tm) can be expressed on the cell surface of WT cells, indicating correct folding of these TLRs ( Fig. 6b,c ). However, with the exception of TLR3tm, none of the other TLRtms could be expressed on the surface of cells that were devoid of either gp96 ( Fig. 6c ) or CNPY3 ( Fig. 6d ). Moreover, we found that gp96 interacted with all other TLRtms, except TLR3tm, by coimmunoprecipitation experiment ( Supplementary Fig. S4 ). The cell surface display assay once again reinforced the notion that gp96 and CNPY3 have shared function in facilitating TLR folding. To further address the roles of CNPY3 in TLR folding, we overexpressed TLR9tm or TLR3tm in HEK293 cells that have a low level of endogenous CNPY3 ( Fig. 7a ), followed by immunoprecipitation of the respective TLRs and their associated molecules. We observed multiple proteins that were coimmunoprecipitated with TLR9tm, but not TLR3tm ( Supplementary Fig. S5 ). These TLR9tm-associated proteins were identified by in-gel trypsin digestion and mass spectrometry, which include gp96, as well as multiple other proteins in the ER for protein folding ( Fig. 7b ). Strikingly, when CNPY3 is a limiting factor, there is a clear induction of molecular chaperones by TLR9tm but not by TLR3tm ( Fig. 7c ). Cotransfection of CNPY3 with TLR9tm led to the attenuation of HSP induction ( Fig. 7d ). We conclude that both gp96 and CNPY3 must be present to complete the folding cycle of TLR9 to avoid the overloading and induction of the general molecular chaperone machinery in the ER. 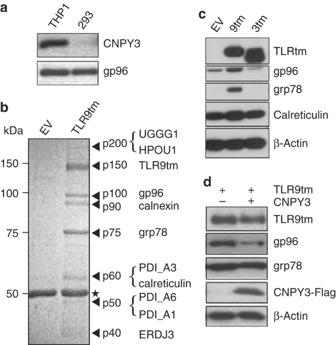Figure 7: Regulation of the general ER chaperone machinery. (a) IB of endogenous CNPY3 and gp96 from THP1 and HEK293 cells. (b) HEK293 cells were transfected with TLR9tm or empty vector (EV). After 48 h, TLR9HA from the total cell lysates was immunoprecipitated with HA antibody. The eluate was resolved on SDS–PAGE and stained with Coomassie blue. Individual bands indicated by arrows were cut, trypsin-digested and sequenced by mass spectrometry. The identities of p40-p200 are indicated. The asterisk represents Ig heavy chain. (c) HEK293 cells were transfected transiently with empty vector (EV), TLR9tm (9tm) or TLR3tm (3tm) expression vector, followed by IB, for indicated proteins. (d) HEK293 cells were transfected with TLR9tm or a combination of TLR9tm and CNPY3 expression vector, followed by IB for indicated proteins. Figure 7: Regulation of the general ER chaperone machinery. ( a ) IB of endogenous CNPY3 and gp96 from THP1 and HEK293 cells. ( b ) HEK293 cells were transfected with TLR9tm or empty vector (EV). After 48 h, TLR9HA from the total cell lysates was immunoprecipitated with HA antibody. The eluate was resolved on SDS–PAGE and stained with Coomassie blue. Individual bands indicated by arrows were cut, trypsin-digested and sequenced by mass spectrometry. The identities of p40-p200 are indicated. The asterisk represents Ig heavy chain. ( c ) HEK293 cells were transfected transiently with empty vector (EV), TLR9tm (9tm) or TLR3tm (3tm) expression vector, followed by IB, for indicated proteins. ( d ) HEK293 cells were transfected with TLR9tm or a combination of TLR9tm and CNPY3 expression vector, followed by IB for indicated proteins. Full size image There are several well-characterized molecules that serve specifically as HSP90 cochaperones, including HOP, p23, AHA1, CDC37, FKBP-52 and UNC45, to facilitate client protein folding [9] , [38] . In contrast, gp96 cochaperones have not been discovered, leading to a long-held notion in the field that this chaperone has a unique and cochaperone-independent mode of mechanism of action. This is perplexing, given the structural evidence that ATP binding alone is not enough to induce a favourable change of the gp96 conformation to facilitate client protein folding [5] , [39] . Although the post-translational regulation of TLRs by both gp96 and CNPY3 has been revealed previously, no study has linked the function of these two proteins together. In this study, we have demonstrated for the first time that CNPY3 is a TLR-specific cochaperone of gp96, on the basis of biochemical, genetic and functional evidence. Specifically, we show the following: (i) deletion of either gp96 or CNPY3 results in indistinguishable post-translational inactivation of multiple TLRs, except TLR3; (ii) gp96 and CNPY3 colocalize in the ER compartment; (iii) gp96 and CNPY3 directly interact with each other, and that interaction is sensitive to adenosine nucleotide; (iv) the interaction between gp96 and CNPY3 was demonstrated in multiple cell types. Moreover, gp96 and CNPY3 are present in the same high-molecular-weight complex with TLR9; (v) disruption of the interaction between gp96 and CNPY3 by a point mutation of either the gp96 N domain (E103A) or CNPY3 (M145K) results in loss of TLR9 function; (vi) gp96–TLR9 interaction is dependent on the presence of CNPY3; (vii) CNPY3 does not interact efficiently with TLR9 in the absence of gp96; (viii) TLR9 cleavage and maturation did not occur in the absence of either gp96 or CNPY3 and; (ix) in the absence of CNPY3, overexpression of the TLR9 ectodomain strongly induces protein chaperones in the ER. Our conclusion explains the complete phenocopy of TLR defects in gp96 KO- [10] and CNPY3-null mice [25] , [28] , and it is consistent with the fact that these two molecules are colocalized in the ER lumen, coexpressed in multiple cell types and codistributed phylogenetically. The requirement for cochaperones in folding client proteins by gp96 is unexpected and novel, and our study thus represents a significant advancement in the field of HSP90 biology. By sequential immunoprecipitation and gel filtration, we have demonstrated that TLR9 is present in the high-molecular-weight complex that contains both gp96 and CNPY3. The ternary complex was also confirmed by coimmunoprecipitation from all three directions. However, the stoichiometry of this interaction remains unclear. Both TLR9 and gp96 are known to form dimers. CNPY3 may also homodimerize or oligomerize. Thus, the TLR, gp96 and CNPY complex could be at 2:2:2 ratio, making the size of the complex reach at least ∼ 600 kDa, which is consistent with our gel filtration data. The precise roles of CNPY3 in assisting the gp96-dependent step of TLR folding also require further experimentation. It is, however, revealing to consider our data in the context of the known gp96 structure. The function of gp96 in folding TLRs is dependent on both ATP binding and ATPase activity [11] , [40] . The structure of the near full-length gp96 dimer in complex with AMP-PNP and ADP revealed an identical twisted 'V'-shape conformation with closed C domains and open N domains in opposing orientation [5] . This conformation most likely reflects a relaxed low-energy state of gp96. Thus, ATP binding of gp96 does not drive it into a hydrolytically productive conformation because of the open N domain and relaxed N–M orientation, which leaves the critical residue R448 for the ATPase activity of gp96 too distant from the γ phosphate of the ATP. The structural study of gp96 thus argues strongly for additional accessory molecules for gp96 to complete its chaperone cycle. We found that CNPY3 binds to the N domain of gp96 (N355) and this binding is lost with a single E103A mutation or in the presence of ATP. These data support the contention that CNPY3 binds to the region in the N domain close to the ATP-binding pocket of gp96. Similar to the action of cdc37 for HSP90 (refs. 41 , 42 ), by binding to the ATP-free N domain of gp96, CNPY3 likely keeps gp96 in the relaxed state to allow 'loading' of substrates onto the free gp96. Although speculative, this idea is consistent with our observation that CNPY3–gp96 interaction is critical for their binding to TLR9. The binding of substrates likely then induces further conformational changes of the gp96 N domain, resulting in an ATPase-dependent folding of bound substrates. Our work, however, does not exclude the functions of CNPY3 by itself in folding other gp96-independent protein substrates. Equally important, CNPY3 is not required for gp96 in folding the entirety of the gp96 clientele. For example, gp96 is also a molecular chaperone for select integrins, including α4 and β2 [11] , [12] . However, this function of gp96 does not depend on CNPY3, as integrin expression is normal in CNPY3 KO cells [25] . In addition, we demonstrated that gp96 E103A was unable to complex with CNPY3, and thus lost its TLR chaperone function. Yet, gp96 E103A retains its ability to chaperone integrins. Taken together, the cochaperone property of CNPY3 for gp96 is substrate specific. There are many precedents for client protein-specific cochaperones of HSP90, including CDC37 for the folding of kinases [42] , FKBP-52 for steroid receptors [43] and UNC45 for myosin [44] . The structural basis by which TLR3 and TLR9 have a dramatic difference in their requirement for gp96/CNPY3 remains unclear. As TLR3 is heavily glycosylated [45] , one possibility would be that the glycosylation of TLR3 alone serves as an effective chaperoning mechanism, relegating it somewhat independent of additional protein chaperones. Another possibility that is yet to be ruled out is the presence of TLR3-unique chaperone(s) that replaces the function of gp96 and CNPY3. Our data allow us to propose the following model on the coordinated roles of gp96 and CNPY3 in the step-wise folding of TLR9 ( Fig. 8 ). We believe that the initial folding and glycosylation of nascent TLR9 (TLR9 precursor 0) is mediated by the conventional glycoprotein folding machinery, including the CNX and calreticulin cycle and other ER chaperones such as grp78 and gp96. The role of gp96 in the initial folding of nascent TLR9 is not dependent on CNPY3, but rather represents a component of the general ER protein folding machinery [6] , [46] , [47] . Neither gp96 nor CNPY3 alone is able to fold TLRs to their full maturation status. As the binding of TLR9 by CNPY3 and gp96 is dependent on each other, we suggest that the CNPY3-gp96 interaction is essential for adopting a favourable conformation of both proteins in order to bind and fold TLR9 in the ER. Only fully folded TLR9 (TLR9 precursor 2) then translocates to the endolysosome with the aid of unc93b [16] . In the acidic environment, TLR9 then fully matures into a functional receptor through the proteolytic cleavage of the N-terminal 14 LRRs by cathepsins [17] , [18] or other proteases [48] . 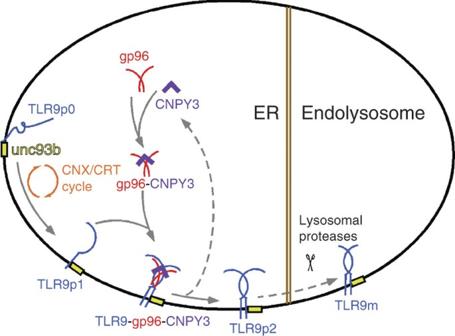Figure 8: A model for the coordinated roles of ER chaperones in TLR9 folding. The initial folding and glycosylation of nascent TLR9p0 (TLR9 precursor 0) are mediated by the ER general glycoprotein-folding machinery, including calnexin (CNX) and calreticulin (CRT). CNPY3 and gp96 must form a complex to more efficiently interact with TLR9p1 (TLR9 precursor 1). gp96–CNPY3 accelerates the tertiary folding of TLR9. Folded TLR9p2 (TLR9 precursor 2) then dissociates from the gp96–CNPY3 complex and translocates to the endolysosome with the aid of the membrane protein unc93b. TLR9 completes its maturation cycle after proteolytic cleavage of the first N-terminal 14 LRRs in the endolysosome. Dotted line represents steps that are not fully characterized. Figure 8: A model for the coordinated roles of ER chaperones in TLR9 folding. The initial folding and glycosylation of nascent TLR9p0 (TLR9 precursor 0) are mediated by the ER general glycoprotein-folding machinery, including calnexin (CNX) and calreticulin (CRT). CNPY3 and gp96 must form a complex to more efficiently interact with TLR9p1 (TLR9 precursor 1). gp96–CNPY3 accelerates the tertiary folding of TLR9. Folded TLR9p2 (TLR9 precursor 2) then dissociates from the gp96–CNPY3 complex and translocates to the endolysosome with the aid of the membrane protein unc93b. TLR9 completes its maturation cycle after proteolytic cleavage of the first N-terminal 14 LRRs in the endolysosome. Dotted line represents steps that are not fully characterized. Full size image In conclusion, we have uncovered a sophisticated mechanism of TLR folding in the ER that depends on gp96 and its cochaperone CNPY3. The mutual dependence of gp96 and CNPY3 is restricted to the folding of TLRs but not integrins. Neither gp96 nor CNPY3 alone is able to chaperone TLRs. Further studies are imperative to understand the regulation of the gp96–CNPY3 interaction, including the site, duration and affinity of their interaction, the precise roles of CNPY3 in regulating other aspects of gp96 function and to identify additional cochaperones and mechanisms of gp96 for folding non-TLR client proteins. Mice and cell lines hsp90b1 flox mice and Mφ-specific gp96 KO mice were described previously [10] . tlr2 −/− tlr4 −/− mice were generated in-house by intercrossing respective single KO mice. tlr3 −/− mice [22] were obtained from A. Vella (University of Connecticut). All mice were kept in specific pathogen-free conditions and handled in accordance with the National Institutes of Health federal guidelines. gp96-mutant and WT pre-B cell lines were provided by B. Seed (Harvard University). HEK293FT cells were purchased from Invitrogen. Phenoix-Ecotropic retrovirus packaging cells were obtained from A. Adler (University of Connecticut). Constructs pUNO vectors expressing C-terminal HA-tagged mouse TLR complementary DNAs (pUNO-mTLR-HA), including TLR3, TLR4, TLR9 and TLR11, were purchased from Invivogen. To generate TLR9HA retrovector, we amplified TLR9HA from pUNO-TLR9HA and inserted it between Bgl II and Eco RI cloning sites on MigR and BLR. The pDisplay vector was purchased from Invitrogen. The surface expression of TLRtm was monitored by antibody against the HA epitope embedded immediately after the signal peptide in the engineered chimeras. The ectodomains of TLR3 (aa 26–705), TLR4 (aa 26–638), TLR9 (26–819) and TLR11 (22–709) were subcloned into pDisplay and were designated as TLRtm constructs. The TLRtm expression cassettes were further subcloned into MigR to generate MigR-TLRtm. pLentiCNPY3 shRNA vector was constructed using the pLL3.7 vector, targeting the 5′-GAGTTTGAAGAGGTGATTGAG-3′ sequence of murine CNPY3 and propagated using 293 FT cells (ATCC). The GST-tagged complete coding sequence of murine CNPY3 complementary DNA was PCR amplified and cloned into pGEX plasmid (GE Healthcare). Quantitative-polymerase chain reaction Total RNA was extracted with the NucleoSpin RNA II kit according to the manufacturer's protocol (Clontech). The mRNA was reverse transcribed with Superscript II (Invitrogen). Complementary DNA was quantified by quantitative-polymerase chain reaction (Q-PCR) with Bio-Rad iCycler. Q-PCR data were analysed with the corresponding software, and the number of PCR cycles to reach the threshold of detection ( C t ) was calculated. Samples were run in duplicates. β-Actin was used as an internal control. The primer sequences of CNPY3 are as follows: forward, 5′-AAAGGACACGAGTTGCCTAGCAGA-3′; reverse, 5′-TCTGCTAGGCAACTCGTGTCCTTT-3′. Antibodies and enzyme-linked immunosorbent assay Lipopolysaccharide (from Escherichia coli , serotype O55:B5), brefeldin A, phorbol 12-myristate-13-acetate, radicicol and ionomycin were purchased from Sigma-Aldrich. polyI:C, R848, CpG and GpC were obtained from Invivogen. CNPY3 stealth small interfering RNA oligos (5′-CCCGCUGCCUCUUAUUUCCUUUGCU-3′) and control oligo (5′-CCUGCCUCUUAUUUCCUUUGCGCU-3′) were obtained from Invitrogen. Glutathione sepharose 4B was purchased from GE Healthcare. Glutathione was obtained from Sigma-Aldrich. The antibodies used in this study were reactive to gp96 (9G10) and grp78 (Stressgen), gp96 (Everest), CNX (Santa Cruz Biotechnology), FLAG epitope and β-actin (AC-74) (Sigma-Aldrich), HA (16B12) (Covance), GST (GenScript), IL-6, tumour-necrosis factor-α, TLR2 and CD69 (eBiosciences) and CNPY3 (Sigma-Aldrich). Cytokine levels were measured using ELISA kits from BD Biosciences according to the manufacturer's protocol. Protein purification and in vitro binding and ATPase assay gp96 was purified from mouse livers using an established method [3] , which consists of cell fractionation, ultracentrifugation, Con A-Sepharose and DEAE chromatography. GST and GST-tagged mouse CNPY3-GST were expressed in E. coli and purified by glutathione-affinity chromatography. DnaK was removed by ADP-agarose column (Sigma-Aldrich). An enzyme-linked immunosorbent assay (ELISA)-based method was used to determine whether CNPY3 directly interacts with gp96. In brief, a 96-well ELISA plate was coated with CNPY3-GST or GST overnight, followed by blocking with 3% bovine serum albumin, and washing and incubation with different concentrations of gp96 in the presence or absence of ATP, ADP, AMP-PNP and radicicol at room temperature for 2 h. The plate was then washed and incubated with a rabbit gp96 antibody, followed by treatment with an HRP-conjugated secondary antibody. After a thorough wash, the plate was developed with tetramethylbenzidine substrate solution and the optical density was read at 450 nm. The ATPase activity of gp96 with and without CNPY3 was performed using γ-p 32 -ATP as described [49] . Flow cytometry Surface staining of cells and flow cytometry were carried out as described [10] , [36] . To stain intracellular cytokines, cells were fixed in 4% paraformaldehyde and permeabilized in 0.25% saponin. Cells were acquired on FACS Calibur (Becton Dickinson) and results were analysed with FlowJo software (Tree Star). Immunoblot Cells were washed twice in cold phosphate-buffered saline (PBS), pelleted and lysed in RIPA buffer (1% NP40, 1% sodium deoxychloate, 0.1% sodium dodecyl sulphate (SDS), 150 mM NaCl, 2 mM EDTA, 0.01 M sodium phosphate pH 7.2 supplemented with protease inhibitor cocktail). Protein concentration of the postnuclear lysate was quantified by Bradford assay (BioRad). Samples were denatured by mixing with SDS loading buffer and dithiothreitol, heated at 95°C for 5 min and spun to remove pellets. Samples were run on 10% SDS–polyacrylamide gel electrophoresis, and transferred onto polyvinylidene difluoride membrane after electrophoresis. The membrane was blocked with 5% milk/PBS, followed by sequential incubation with primary antibody and horseradish peroxidase-conjugated secondary antibody. After extensive washing, the membrane was soaked in substrate solution (Pierce) for 5 min. Luminescent signals were recorded on X-Omat LS film. Immunoprecipitation and gel filtration Unless otherwise indicated, cells were treated with 0.5 mM dithiobis succinimidyl propionate for 30 min, followed by lysis in RIPA buffer. An equal amount of lysate was precleared with protein G beads for 4 h. Precleared lysates were further incubated with anti-HA monoclonal antibody/protein G beads at 4°C overnight. The antibody–bead complexes were then extensively washed with RIPA buffer. The bound proteins were eluted by heating the beads at 95°C in reducing SDS-loading buffer. For mass-spectrum analysis, sequential immunoprecipitation and gel filtration, the bound proteins were eluted by incubating with HA peptide (Sigma-Aldrich) at 37°C for 15 min. For gel filtration, the complex was resolved on a Superdex-200 10/300 GL column (GE Healthcare) at a flow rate of 0.5 ml min −1 and fractions were collected on a volume base (0.5 ml per tube) throughout the chromatogram. Each fraction was concentrated and visualized by SDS–polyacrylamide gel electrophoresis, followed by immunoblotting. The column was calibrated by performing an identical chromatographic separation with a mixture of molecular mass standards (Bio-Rad). Transfection To express epitope-tagged TLRs ectopically in HEK293 cells, cells were transfected with TLRtm or CNPY3 expression vector using lipofectamine 2000 (Invitrogen) according to the manufacturer's protocol. WT and gp96 mutant pre-B cells [11] were transiently transfected with pUNO-TLR-HA by nucleotransfection (Amaxa). Retroviral transduction Cells were seeded in a 24-well plate and cultured in fresh complete growth medium. One day later, cells were spin-infected with recombinant retrovirus (1000 g , 32°C, 90 min) in a desktop centrifuge. In-gel digestion and LC-MS/MS analysis This was performed as previously described without significant modifications [50] . Trypsin-digested proteins were analysed using a linear ion trap mass spectrometer (Finnigan LTQ, Thermo Finnigan). Samples were loaded onto a 10-cm×100-μm capillary C18 reverse-phase column by a microautosampler (Famos, Dionex), followed by LC-MS/MS (liquid chromatography-mass spectrometry-tandem mass spectrometry) analysis on the LTQ. The mass spectrometry data file was searched against the current human protein database. Immunofluorescence microscopy CNPY3-FLAG-transduced Raw264.7 cells were seeded and cultured on glass coverslips at 37°C overnight, washed with 1× PBS, fixed immediately with 4% paraformaldehyde, permeablized with 100% cold methanol and blocked for 60 min in 5% normal goat serum. Cells were stained sequentially with gp96 antibody, Alexa Fluor-488 goat antirat antibody (gp96, green), mouse anti-FLAG antibody and Alexa Fluor-594 (CNPY3, red). Nuclei were counterstained with 4,6-diamidino-2-phenylindole. Isotype control antibody was also used to ensure specificity (data not shown). Samples were mounted onto glass slides with a mounting medium (Biomedia) to retard photobleaching, sealed with nail enamel and imaged with a Zeiss LSM 510 Axiovert 100 confocal microscope equipped with an argon/krypton laser (Zeiss). Statistical analysis Student's t -test was used for statistical analysis. Values of P <0.05 were considered to represent statistically significant differences. How to cite this article: Liu, B. et al . Folding of Toll-like receptors by the HSP90 paralogue gp96 requires a substrate-specific cochaperone. Nat. Commun. 1:79 doi: 10.1038/ncomms1070 (2010).